Bio-optimized energy transfer in densely packed fluorescent protein enables near-maximal luminescence and solid-state lasers Bioluminescent organisms are likely to have an evolutionary drive towards high radiance. As such, bio-optimized materials derived from them hold great promise for photonic applications. Here, we show that biologically produced fluorescent proteins retain their high brightness even at the maximum density in solid state through a special molecular structure that provides optimal balance between high protein concentration and low resonance energy transfer self-quenching. Dried films of green fluorescent protein show low fluorescence quenching (−7 dB) and support strong optical amplification ( g net =22 cm −1 ; 96 dB cm −1 ). Using these properties, we demonstrate vertical cavity surface emitting micro-lasers with low threshold (<100 pJ, outperforming organic semiconductor lasers) and self-assembled all-protein ring lasers. Moreover, solid-state blends of different proteins support efficient Förster resonance energy transfer, with sensitivity to intermolecular distance thus allowing all-optical sensing. The design of fluorescent proteins may be exploited for bio-inspired solid-state luminescent molecules or nanoparticles. There is an increasing interest in using biologically derived or even biologically produced materials and structures for photonic applications. Such materials provide excellent environmental compatibility and show good biocompatibility in medical applications. Developed by nature in a multi-million year evolutionary process, biologically produced materials frequently make use of ingenious concepts that provide characteristics superior to synthetic or inorganic materials. So far, research efforts in this field have been mostly concerned with passive, light-manipulating structures, including iridescent scales of butterfly wings for trace solvent sensing [1] and infra-red detection [2] , use of silk protein for biocompatible optical waveguides [3] , photoreceptor-based achromatic quarter-wave retarders [4] and many others. Beyond these passive optical materials and structures, however, is the less-well-explored field of natural active light emitters based on biomaterials [5] . Recently, we have reported on the use of mammalian and bacteria cells that express enhanced green fluorescent protein (eGFP) as living sources of laser light [6] , [7] . While these lasers will be useful for cellular sensing [8] and to develop self-healing laser sources, a solid-state system would offer advantages in practicality for many settings. A number of different types of fluorescent proteins (FPs) are found in nature in organisms such as the Aequorea victoria jellyfish, the Renilla reniformis sea pansy and multiple reef corals. During the evolutionary process, FPs have evolved to form the acceptor part of a Förster resonance energy transfer (FRET) pair in the light-emitting organs of several bioluminescent organisms. Many naturally occurring FPs occur as dimers or tetramers [9] , [10] . There is evidence that FPs constitute several percent of the total mass of the photogenic cells in bioluminescent organisms [11] , [12] . Within these cells, the FP molecules are localized to the membrane of submicrometre-sized organelles [13] , [14] , and we, therefore, expect the local concentration at the membrane to exceed 20% by mass. Here, we show that the condensed solid-state form of FPs offers excellent optical properties; in particular, bright fluorescence, high optical gain, lasing capability and, interestingly, a characteristic sensitivity to external stimuli, such as humidity, that can alter the intermolecular spacing. Moreover, the efficient solid-state fluorescence enables FRET processes between neighbouring molecules in blends of two different FPs without the need for molecular linkers. Fluorescence from dry-condensed eGFP The actual fluorophore of FPs is enclosed by a nano-cylinder that consists of eleven β-sheets and that is about 2.4 nm in diameter and 4.2 nm in height ( Fig. 1a ; refs 15 , 16 ). This protective shell (β-barrel) acts as natural ‘bumper’ and prevents close contact between fluorophores of neighbouring FPs ( Fig. 1b ). We suspect that the geometrically enforced separation between fluorophores limits intermolecular energy migration even at the highest possible concentration ( Fig. 1c ) and thus reduces luminescence quenching. Without the β-sheet shell, dense aggregation of fluorophores would result in excessive quenching ( Fig. 1d ). 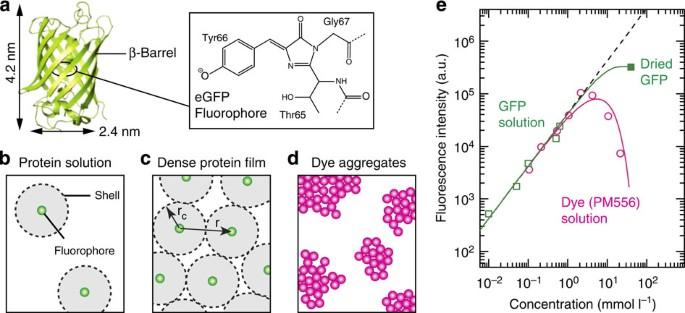Figure 1: Biologically produced fluorescent proteins are resistant to self-quenching of fluorescence in solid state. (a) Protein structure of enhanced green fluorescent protein (eGFP) comprising of a nano-cylinder (β-barrel) enclosing the active fluorophore in the centre. Inset: the hydroxybenzylidene–imidazolidinone fluorophore of eGFP. (b) Schematic illustration of eGFP molecules in diluted protein solution, and (c) of densely packed protein film where fluorophores remain separated by a distance of at least 2rcthus reducing self-quenching. (d), The fluorophores of synthetic dyes tend to collide or aggregate at high concentration, leading to quenching by unproductive donor–donor transfer. (e) Fluorescence intensity of aqueous eGFP solutions (open squares) with different concentrations and of a thin film of solid-state eGFP (at 40 mmol l−1, filled squares). Fluorescence of a synthetic pyrromethene dye (open circles). All data normalized to sample thickness and corrected for excitation depletion (see Methods). Black dashed line, linear fit at low concentration (with no concentration quenching). Green and pink lines, Förster-type quenching model for eGFP and aggregation-induced quenching model for pyromethene dye, respectively. Figure 1: Biologically produced fluorescent proteins are resistant to self-quenching of fluorescence in solid state. ( a ) Protein structure of enhanced green fluorescent protein (eGFP) comprising of a nano-cylinder (β-barrel) enclosing the active fluorophore in the centre. Inset: the hydroxybenzylidene–imidazolidinone fluorophore of eGFP. ( b ) Schematic illustration of eGFP molecules in diluted protein solution, and ( c ) of densely packed protein film where fluorophores remain separated by a distance of at least 2 r c thus reducing self-quenching. ( d ), The fluorophores of synthetic dyes tend to collide or aggregate at high concentration, leading to quenching by unproductive donor–donor transfer. ( e ) Fluorescence intensity of aqueous eGFP solutions (open squares) with different concentrations and of a thin film of solid-state eGFP (at 40 mmol l −1 , filled squares). Fluorescence of a synthetic pyrromethene dye (open circles). All data normalized to sample thickness and corrected for excitation depletion (see Methods). Black dashed line, linear fit at low concentration (with no concentration quenching). Green and pink lines, Förster-type quenching model for eGFP and aggregation-induced quenching model for pyromethene dye, respectively. Full size image To verify this prediction quantitatively, we investigated solutions of recombinant eGFP. eGFP has similar molecular dimensions and structure to the wild-type FP in Aequorea victoria but improved light absorption. The fluorescence intensity was measured over a range of concentrations from micro- to millimolar and also for a thin film of solid-state eGFP ( Fig. 1e ). The latter has a nominal concentration of ~40 mmol l −1 . As a reference, the same experiment was performed with a state-of-the-art synthetic green-fluorescing pyrromethene dye (disodium-1,3,5,7,8-pentamethylpyrromethene-2,6-disulfonate-difluoroborate, molecular mass 466 Da). The extinction coefficients ( ε ) and the fluorescence quantum yields ( QY ) in dilute aqueous solution are similar for eGFP and for the pyrromethene dye: ε 488 nm =5.6 × 10 4 l mol −1 cm −1 , QY =60-70% for eGFP [17] and ε 488 nm =6.1 × 10 4 l mol −1 cm −1 , QY =73% for the dye. As expected, nearly equal fluorescence intensity was detected for both materials at low concentrations (below 2 mmol l −1 ), linearly increasing with concentration. For higher concentrations, however, the fluorescence from the pyrromethene dye dropped steeply and no fluorescence was detected from solid-state pyrromethene. This phenomenon is known as self-quenching or concentration quenching [18] . By contrast, fluorescence from eGFP increased linearly with concentration for all liquid samples, and, for the solid-state eGFP film, the deviation from the linear trend was measured to be only about −7 dB or a reduction by 80%. A model for intermolecular quenching in fluorescent proteins Previous studies of fluorescence quenching have established that several molecular and photochemical mechanisms contribute to quenching [19] . Static quenching arises when the molecules in the ground state form non-fluorescent complexes (for example, dimers and aggregates). Dynamic quenching is due to a ‘quencher’ that interacts with a molecule in the excited state via electron exchange (Dexter transfer) or FRET and turns off fluorescence. For small-sized organic dyes, static quenching is a major quenching mechanism. Assuming a concentration-dependent aggregation of the dye molecules in pyrromethene solutions ( Supplementary Fig. 1 ), we can reasonably model the dramatic reduction of fluorescence intensity at high concentrations, above several mmol l −1 ( Fig. 1e ). For fluorescent proteins, we suspect that aggregation of fluorophores and short-range collisional quenching, such as electron transfer, are minimal because of the protective β-shell structure. Instead, we expect that the dominant quenching mechanism should involve long-range resonant energy transfer to quenchers, which are most likely eGFP molecules in different non-fluorescent forms. Examples include a small fraction of proteins that suffer from misfolding in E. coli or from denaturation and have fluorophores capable of absorbing in the blue/green part of the spectrum but are non-fluorescent [20] . Other potential candidates include direct resonant excitation of nonradiative pathways (energy levels) in a neighbouring eGFP without going through the excited state of the fluorophore. We developed a simple theoretical model that describes this general quenching mechanism by introducing a loss parameter ε ( ≪ 1), which is the ratio of the probability for resonant energy transfer to a quencher versus the probability of transfer to an active fluorophore ( Supplementary Discussion 1 ). We define an effective quenching radius R Q : where N is the effective number of acceptor proteins in the neighbourhood, and R F is the Förster radius between two fluorophores. The fluorescence efficiency ( η ) depends on the fluorophore-to-fluorophore distance ( r ) as The fluorescence intensity ( I ) is given by , where A is a proportionality constant, c is concentration, and ρ ( r ) is the nearest-neighbour distribution function [21] , [22] , which gives the probability density of a molecule to be separated from its nearest neighbour by a distance r . eGFP was modelled as a hard sphere with a diameter ( R ) of 3.3 nm, that is, ρ ( r )=0 for r < R due to geometrical hindrance ( Supplementary Fig. 2 ). Our experimental data can be described reasonably well with this model, using ε =0.04–0.05 and R F =4.65 nm (derived from the emission and absorption spectra of eGFP, Methods), and N =1–12 increasing linearly with concentration ( Fig. 1e ). According to this analysis, R Q varies from 2.8 at the lowest concentration ( c →0) to 4.2 nm at the highest concentration ( c =40 mmol l −1 ). The fluorescence intensity of solid state or very highly concentrated FP can be approximated by using c = V / R 3 and ρ ( r )= δ ( r − R ) with V as proportionality factor. The intensity reaches a rather sharp maximum when the protein size R corresponds to R Q ( Supplementary Fig. 3 ). Interestingly, the actual size of individual FP molecules indeed happens to be close to the theoretical optimum for maximum brightness at high concentration. Optical gain and amplified spontaneous emission Due to its favourable fluorescence properties and the large number of active molecules per volume, we expect solid-state eGFP to provide large optical gain. This was tested by measuring the amplified spontaneous emission (ASE) from a thin eGFP film (thickness, 400 nm). The films were excited with ns-pulses of 485 nm light that were focused to a stripe on the sample surface. The emission from the film was collected at the edge of the substrate ( Fig. 2a , Methods). This excitation geometry supports optical amplification of spontaneously emitted photons that propagate through the film along the direction of the excitation stripe. As the energy of the excitation pulses is increased, this ASE should begin to dominate over omnidirectional spontaneous emission. As a result, the emission from the edge of the substrate will increase super-linearly in intensity and decrease in spectral width [23] . A dramatic reduction in the spectral width of the collected light was indeed observed once the excitation flux ( F p ) was increased beyond ~1.5 mJ cm −2 ( Fig. 2b ). This was accompanied by a threshold-type increase in output intensity ( Fig. 2c ). To quantify the net optical gain coefficient ( g ) within the eGFP film, the output intensity ( I ) was measured as a function of the excitation stripe length on the sample ( x ) ( Fig. 2d ). 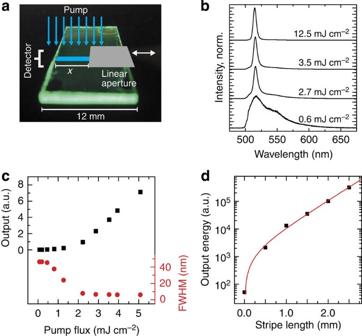Figure 2: Amplified spontaneous emission (ASE) in slab waveguides formed by thin films of enhanced green fluorescent protein (eGFP). (a) Picture of eGFP film on glass substrate with schematic illustration of the ASE measurement. Length of excitation stripe on the film (x) is adjusted by a linear aperture. (b) Emission spectrum collected by detector for different pump fluxes. (c) Energy of ASE pulses (top) and spectral width of ASE (bottom) as a function of pump flux for a 3 mm long excitation stripe. (d) Energy of ASE pulses as a function of length of excitation stripe for an excitation flux of 9 mJ cm−2. Red line, fit to gain equation. norm., normalized. The data were fitted with the gain equation [24] : Figure 2: Amplified spontaneous emission (ASE) in slab waveguides formed by thin films of enhanced green fluorescent protein (eGFP). ( a ) Picture of eGFP film on glass substrate with schematic illustration of the ASE measurement. Length of excitation stripe on the film ( x ) is adjusted by a linear aperture. ( b ) Emission spectrum collected by detector for different pump fluxes. ( c ) Energy of ASE pulses (top) and spectral width of ASE (bottom) as a function of pump flux for a 3 mm long excitation stripe. ( d ) Energy of ASE pulses as a function of length of excitation stripe for an excitation flux of 9 mJ cm −2 . Red line, fit to gain equation. norm., normalized. Full size image Here, B is a proportionality factor relating the spontaneous emission in the film to F p . For F p =9 mJ cm −2 , we obtain g =22 cm −1 or 96 dB cm −1 . Although substrate, film thickness and fabrication process were not optimized for low optical loss, this value is on par with the gain achieved in synthetic hydrocarbon-based gain materials [25] and indicates that solid-state eGFP is a promising candidate for providing optical gain in lasers. A single-mode solid-state protein laser To demonstrate lasing from solid-state protein, a vertical cavity surface emitting laser (VCSEL) was fabricated that comprised a thin film of eGFP sandwiched between two distributed Bragg mirrors with reflectivity >99.9% in the 500–560 nm range ( Fig. 3a ). The structure was pumped by a compact, passively q-switched microchip laser (pulse duration 2 ns; repetition rate 100 Hz; λ =473 nm). 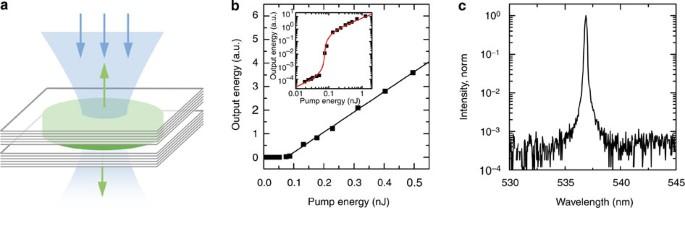Figure 3: Vertical cavity surface emitting laser (VCSEL) based on solid-state fluorescent protein. (a) Schematic of VCSEL comprising a thin layer of enhanced green fluorescent protein (eGFP) as gain material sandwiched between two highly reflective Bragg mirrors. (b) Output of eGFP VSCEL versus pump pulse energy (filled squares). Line, linear fit. Inset: Fit to the same data using rate equation model, shown on log–log scale. (c) Output spectrum of VCSEL structure pumped above threshold. norm., normalized. Figure 3b shows the energy of the light pulses emitted by the structure for different pump pulse energies ( E p ). Above a pump threshold of E p =82 pJ, the output power increased steeply with pump energy. When plotting the input–output characteristics on a log–log scale, two linear regimes of operation become apparent, associated with spontaneous emission and stimulated coupling to the laser mode, respectively ( Fig. 3b , inset). The input–output characteristics are well described using a simple rate equation approach [26] , yielding a spontaneous emission factor of the populated cavity mode of β =2.6 × 10 −4 . The eGFP VCSEL operates in single longitudinal and transverse mode, with a spectral linewidth below the spectrometer resolution (full width at half maximum (FWHM) <0.06 nm) and side-band suppression better than the dynamic range of the detector (~35 dB; Fig. 3c ). The clear threshold behaviour and the spectral narrowing are unambiguous evidence for lasing. Due to the increased concentration, solid-state eGFP provides much higher gain per unit length than eGFP solutions leading to thresholds >100-fold lower than in previous reports on solution-based eGFP lasing [6] . In terms of absolute threshold energy, the eGFP VCSEL outperforms organic semiconductor lasers with similar microcavity architectures [27] . Figure 3: Vertical cavity surface emitting laser (VCSEL) based on solid-state fluorescent protein. ( a ) Schematic of VCSEL comprising a thin layer of enhanced green fluorescent protein (eGFP) as gain material sandwiched between two highly reflective Bragg mirrors. ( b ) Output of eGFP VSCEL versus pump pulse energy (filled squares). Line, linear fit. Inset: Fit to the same data using rate equation model, shown on log–log scale. ( c ) Output spectrum of VCSEL structure pumped above threshold. norm., normalized. Full size image ‘Protein-stain’ ring lasers In addition to providing optical gain, we reasoned that FPs can enable facile self-assembly into optical ring resonators, thus allowing generation of laser light without an external mirror-based cavity. Instead, the optical feedback is provided by a protein ring resonator on a transparent substrate. The fabrication is based on the ‘coffee-stain’ effect [28] : When a drop of a solution dries on a surface, capillary flow during solvent evaporation deposits non-volatile components in the solution at the outer edge of the drop. We found that microlitre-droplets of eGFP solution (100 μmol l −1 ) form very homogeneous rings of protein with sizes of 0.5–2 mm in diameter and with uniform width and thickness of a few micrometres ( Fig. 4a,b ). We estimated the refractive index of dried eGFP to be n ≈1.51 ( Supplementary Fig. 4 ), in agreement with the literature [29] . When deposited on a low refractive-index substrate ( n substrate ≈1.34, Methods and ref. 30 ), the ‘protein stains’ are therefore expected to serve as waveguides by total internal reflection and to support whispering gallery modes. 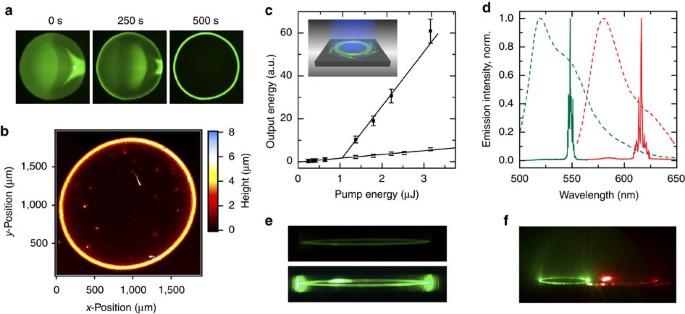Figure 4: Protein ring resonator laser fabricated by coffee-stain effect-based self-assembly. (a) Fluorescence images of droplet (volume, 0.5 μl) of enhanced green fluorescent protein (eGFP) solution (concentration, 100 μmol l−1) on a low refractive-index substrate at different times during drying of droplet. (b) Surface topography of ‘protein stain’, acquired by optical profilometry. (c) Output energy of eGFP ring resonator as function of pump energy for the intact resonator (filled squares) and after the ring was cut open (open squares). Lines, linear fits. Inset illustrates pumping configuration (blue beam) and tangential light-leakage from ring resonator (green arrows). (d) Emission spectra of eGFP (green line) and tdTomato (red line) ring laser below (dashed lines) and above (solid lines) threshold. (e) Images of ring laser output below threshold (0.5 μJ, top) and above threshold (3 μJ, bottom). (f) Spatially controlled droplet deposition enables fabrication of multi-colour arrays of self-assembled ring lasers. The diameters of the protein rings ineandfwere ~1 mm. norm., normalized. Figure 4: Protein ring resonator laser fabricated by coffee-stain effect-based self-assembly. ( a ) Fluorescence images of droplet (volume, 0.5 μl) of enhanced green fluorescent protein (eGFP) solution (concentration, 100 μmol l −1 ) on a low refractive-index substrate at different times during drying of droplet. ( b ) Surface topography of ‘protein stain’, acquired by optical profilometry. ( c ) Output energy of eGFP ring resonator as function of pump energy for the intact resonator (filled squares) and after the ring was cut open (open squares). Lines, linear fits. Inset illustrates pumping configuration (blue beam) and tangential light-leakage from ring resonator (green arrows). ( d ) Emission spectra of eGFP (green line) and tdTomato (red line) ring laser below (dashed lines) and above (solid lines) threshold. ( e ) Images of ring laser output below threshold (0.5 μJ, top) and above threshold (3 μJ, bottom). ( f ) Spatially controlled droplet deposition enables fabrication of multi-colour arrays of self-assembled ring lasers. The diameters of the protein rings in e and f were ~1 mm. norm., normalized. Full size image On pumping such a protein ring resonator (diameter, 1.1 mm) from the top, lasing was observed above a threshold of E p =1 μJ, corresponding to a flux of 100 nJ mm −2 ( Fig. 4c ). Figure 4d shows the emission spectrum of the ring laser below and above laser threshold. As in the VCSEL, a collapse of emission linewidth is observed above threshold (FWHM=0.63 nm at E p =3 μJ). Due to the macroscopic size of the ring resonator, a large number of modes contribute to the lasing process, giving rise to a complex emission spectrum. When removing a small segment of the ring (~10° arc) by manual scrubbing, the kink in the input–output characteristics and spectral narrowing were no longer observed, confirming that lasing is indeed from whispering gallery modes ( Fig. 4c , open symbols). A fraction of the light circulating in the ring resonator continuously leaks out, predominantly in the plane of the ring ( Fig. 4c , inset). This leakage is negligible compared with omnidirectional non-guided emission unless the circulating light is amplified by stimulated emission. For sub-threshold pumping, the ring therefore emits uniformly in all directions, whereas, above threshold, the left and right edge of the ring become particularly bright, due to the circulating laser light radiating in tangents to the ring waveguide ( Fig. 4e ). Both the edges are equally bright, which implies bi-directional oscillation. (The additional bright spot in the left upper half of the ring in Fig. 4e is due to scattering from a small defect.) By placing rings of eGFP and tdTomato (a red-emitting FP) next to each other, we achieved simultaneous multi-colour lasing ( Fig. 4d,f ). We envision that the ‘protein stain’ approach may be further developed to create resonators with more complex shapes and functionality and smaller dimensions. This may find applications in integrated photonic devices [31] and microfluidics [32] . All-optical protein ring sensor The ring structure allows us to further investigate the solid-state fluorescence of eGFP. 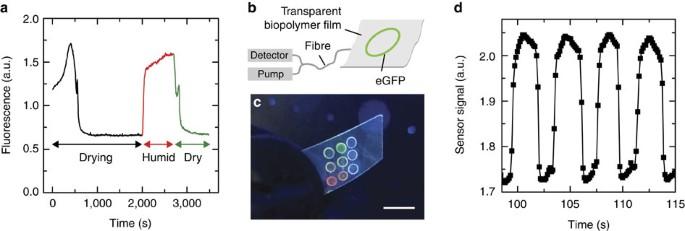Figure 5: Vapour sensitivity of solid-state fluorescent protein. (a) Change in brightness for drying droplet of enhanced green fluorescent protein (eGFP) solution (600 μmol l−1, time 0–2,000 s), recovery of fluorescence in noncondensing water vapour (~90% rel. humidity; 2,000–2,700 s) and partial loss of fluorescence in dry air (2,700–3,500 s). (b) Schematic of proposed integrated sensor based on solid-state fluorescent protein and a biopolymer slab waveguide. (c) Flexible poly(lactic acid) film with rings of different fluorescent proteins in solid-state form, including blue fluorescent protein (BFP), eGFP and tdTomato (scale bar, 5 mm). (d) Fluorescence intensity oscillation over several cycles of exposure to moist and dry air. Figure 5a shows the change in fluorescence intensity collected from the rim of a drying drop of concentrated eGFP solution (600 μmol l −1 ; film thickness ~12 μm). The fluorescence initially increases due to protein accumulation at the rim of the drop. However, past a certain time point, the fluorescence decays rapidly and then stabilizes at ~1/3 of the peak value once the droplet has completely dried. Interestingly, the fluorescence can be fully recovered by exposing the ring to water vapour (~90% rel. humidity, noncondensing), indicating that the effect is associated with the very final stage of drying ( Fig. 5a ). We assume that—upon exposing the protein ring to water vapour—water molecules repopulate the well-ordered stripes of water binding sites on the outside of the β-sheets forming the eGFP cylinder (>50 binding sites in total) [33] . This increases the effective size of the FP molecules and the inter-fluorophore distance and hence considerably reduces self-quenching. (There is a small cavity inside the β-barrel of eGFP housing four additional water molecules. However, as this cavity is closed to the outside [16] , these molecules are unlikely to be released during drying under non-denaturing conditions.) Figure 5: Vapour sensitivity of solid-state fluorescent protein. ( a ) Change in brightness for drying droplet of enhanced green fluorescent protein (eGFP) solution (600 μmol l −1 , time 0–2,000 s), recovery of fluorescence in noncondensing water vapour (~90% rel. humidity; 2,000–2,700 s) and partial loss of fluorescence in dry air (2,700–3,500 s). ( b ) Schematic of proposed integrated sensor based on solid-state fluorescent protein and a biopolymer slab waveguide. ( c ) Flexible poly(lactic acid) film with rings of different fluorescent proteins in solid-state form, including blue fluorescent protein (BFP), eGFP and tdTomato (scale bar, 5 mm). ( d ) Fluorescence intensity oscillation over several cycles of exposure to moist and dry air. Full size image If the protein is integrated on a flexible biocompatible substrate, this effect can form the basis for a bio-integrated sensor. Figure 5b,c show a possible realization of this concept with one or several rings of FP deposited on a film of biocompatible poly(lactic acid). Excitation and readout of the protein were performed by end-fire coupling to the edge of the poly(lactic acid) film, thus using the film as optical waveguide. The kinetics of the brightness change depends on the surface-to-volume ratio of the sample. When exposing a thin ring (thickness ~3 μm; deposited from 50 μmol l −1 eGFP solution) alternately to humidified and dried air, the rise and fall time of the signal were of the order of 250 ms ( Fig. 5d ). FRET in heterogeneous mixture of proteins Pairs of two different FPs can support efficient FRET of excited state energy from one protein molecule (donor) to the other (acceptor). In addition to the 1/ r 6 dependence on intermolecular distance already discussed for transfer between FP molecules of the same type, the FRET efficiency also depends on the overlap between the emission spectrum of the donor and the absorption spectrum of the acceptor. FRET between different proteins with good spectral match (hetero-FRET) is considerably more efficient and occurs over longer distances than FRET between molecules of the same type (provided all other factors are comparable). FRET pairs with a donor–acceptor binding affinity specific to the local biochemical environment are used as optical probes or reporters [34] , [35] . FRET between synthetic dye molecules is an emerging scheme for lasers as it can potentially reduce reabsorption losses and is capable of shifting the pump wavelength to a convenient spectral range [36] , [37] . In solution, a linker between donor and acceptor is used because the average distance between them would otherwise substantially exceed the Förster radius. However, a self-organized solid-state mixture of proteins is expected to provide appropriate distances between donor and acceptor molecules for FRET to occur. We investigated this possibility using blends of eGFP (donor) and tdTomato (acceptor) ( Fig. 6a ). A solution of the two proteins was excited at 473 nm where eGFP is highly absorbing and the absorption of tdTomato is relatively weak. The observed fluorescence was mostly from eGFP; emission from tdTomato was represented only by a weak shoulder in the emission spectrum even for solutions with more tdTomato than eGFP. This is consistent with preferential absorption of the excitation light by eGFP and the absence of energy transfer to tdTomato in solution. In solid state, however, the distance between eGFP and tdTomato molecules is less than their Förster radius (5.0 nm, Methods). Indeed, even a film of eGFP:tdTomato blend that was 7:3 by weight showed stronger emission from tdTomato than from eGFP when excited at 473 nm ( Fig. 6b ). With respect to the solution spectrum of the same blend, the ratio between tdTomato and eGFP emission increased by over 16-fold. Solid-state FRET from eGFP to tdTomato is more efficient than the FRET in conventional peptide-fused donor–acceptor pairs of similar FPs [38] . 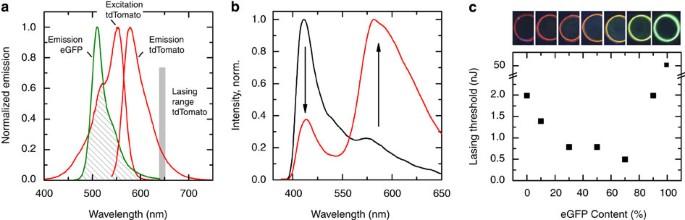Figure 6: Solid-state Förster resonance energy transfer (FRET) between complimentary fluorescent protein molecules. (a) Overlap (dashed area) between emission spectrum of enhanced green fluorescent protein (eGFP) and excitation spectrum of tdTomato, illustrating potential for efficient FRET. Grey bar, wavelength range over which tdTomato shows lasing. (b) Fluorescence spectrum of solution (black line) and solid-state (red line) mixture of eGFP and tdTomato (7:3 by weight) excited within the absorption band of eGFP (λexc=473 nm). (c) Lasing threshold of vertical cavity surface emitting lasers (VCSELs) based on different eGFP:tdTomato blends (0–99% eGFP content). Insets: Fluorescence images of solid-state protein rings of the same eGFP:tdTomato blends under ultraviolet excitation (left to right, increasing eGFP content). norm., normalized. Figure 6: Solid-state Förster resonance energy transfer (FRET) between complimentary fluorescent protein molecules. ( a ) Overlap (dashed area) between emission spectrum of enhanced green fluorescent protein (eGFP) and excitation spectrum of tdTomato, illustrating potential for efficient FRET. Grey bar, wavelength range over which tdTomato shows lasing. ( b ) Fluorescence spectrum of solution (black line) and solid-state (red line) mixture of eGFP and tdTomato (7:3 by weight) excited within the absorption band of eGFP ( λ exc =473 nm). ( c ) Lasing threshold of vertical cavity surface emitting lasers (VCSELs) based on different eGFP:tdTomato blends (0–99% eGFP content). Insets: Fluorescence images of solid-state protein rings of the same eGFP:tdTomato blends under ultraviolet excitation (left to right, increasing eGFP content). norm., normalized. Full size image The effect of FRET is even more pronounced for laser emission from the protein blend. In a laser based on an aqueous solution of eGFP and tdTomato, the threshold for lasing from tdTomato is not affected by the eGFP concentration even when pumping at 473 nm. This indicates that eGFP is not involved in lasing for this configuration. When using a solid-state mixture of the two materials, we do not observe eGFP lasing but detect strong emission ~650 nm, characteristic of tdTomato lasing. The threshold of a laser based on the 7:3 protein blend is four times lower than for pure tdTomato ( Fig. 6c ). Nature has created various wild-type FPs, such as GFP and dsRed, and a variety of derivatives with optimized absorption and emission spectra have been developed. All FPs share the same structural motif with a fluorophore enclosed by a cylindrical β-barrel with nanometre-dimensions. In this work, we have demonstrated that the unique three-dimensional structure of FP molecules allows them to achieve high radiance when condensed to solid state because adjacent fluorophores are separated by approximately their self-quenching radius. This intermolecular distance leads to a good balance between excessive self-quenching and the highest possible packing density and thus offers minimal dead volume. As quenching depends critically on the intermolecular distance (1/ r 6 dependence), such a close agreement in length scales indicates that FPs might have evolutionary evolved for maximal luminescence brightness. Another natural example of tightly controlled chromophore separation is in photosynthesis, where efficient energy transfer to a trap site in light-harvesting complexes is achieved by resonant transfer between chlorophyll molecules with 0.8–1.4 nm separation [39] . A main distinction is, however, that in this case rapid energy loss (‘quenching’) to the reaction centre is the desired endpoint, whereas in the luminescence organs, quenching is a loss to avoid. Therefore, the high packing density of chlorophyll in the light-harvesting units may represent biological optimization for maximal FRET quenching, yet minimal static quenching ( Supplementary Discussion 2 ). In the solid-state form investigated here, the FP molecules are randomly packed and oriented in random directions. We expect that in an ordered state, that is, as a protein crystal, a similar maximal concentration (40 mmol l −1 ) with a comparable level of self-quenching is reached. Unique features of a fluorescent protein crystal, however, are the absence of any light scattering—due to its ordered structure—and the regular alignment of the emissive transition dipole moments of the fluorophores. Therefore, we expect that the device principles demonstrated here can be extended to solid-state protein crystals with the additional advantage of reduced scattering loss. Despite the light scattering loss in randomly stacked solid-state GFP, the dense packing of the fluorophores and the absence of significant quenching results in a high net gain of >22 cm −1 . With a further reduction of scattering and waveguide losses, much higher gains should be achievable (estimating the solid-state gain of eGFP from its absorption coefficient yields g =1,100 cm −1 at 50% inversion). We have also demonstrated that a heterogeneous mixture of two different types of fluorescent proteins in solid state generates effective FRET. According to our model, the FRET efficiency in solid-state FP blends, that is, the probability of an acceptor to emit fluorescence, is given by (including the effect of self-quenching among donors and acceptors): where R F is the effective FRET radius and R Q is the quenching radius of the acceptor ( Supplementary Discussion 3 ). The maximum FRET efficiency occurs at R =( R F R Q ) 1/2 , which is 4–5 nm ( Supplementary Fig. 5 ). The model predicts that the maximum acceptor emission is achieved when the inter-fluorophore distance is approximately equal to R Q , which is 3–4 nm, indicating that the size of FPs indeed results in very favourable separation for maximum FRET-induced fluorescence at high concentration. The model also predicts that in optimized mixtures, acceptor emission can be 10–50 times more intense than the donor emission. By extending our two-protein blends to more complex solid-state mixtures of multiple proteins or of proteins and other functional molecules, we envision that sophisticated functionality can be realized. For example, simultaneous sensing of multiple stimuli that alter the intermolecular distances may be achieved. Coupled with chemically or thermally sensitive polymer substrates, sensing of additional physiologically relevant parameters, such as pH and temperature, would be possible. We believe that the core-shell structure of the fluorescent protein molecule can provide bio-inspiration for other types of fluorescent emitters, such as synthetic organic or inorganic dyes and quantum dots. Light-emitting dendrimers [40] , [41] and core-shell colloidal quantum dots [42] attract increasing levels of interest and indeed already use a structure that resembles the motif of the FP molecule. The study of FPs is expected to direct further optimization of these materials, for example, with respect to controlling multi-exciton Auger recombination, which poses challenges in using quantum dots for lasers [43] , or by guiding the choice of the appropriate generation number of dendrimers to achieve optimal brightness. Recombinant fluorescent protein eGFP was kindly provided by Ji-Joon Song (Korea Advanced Institute of Science and Technology); eGFP was expressed from pET-28a-TEV-eGFP plasmid in Escherichia coli BL21(DE3) RILP. tdTomato was obtained by expression in Escherichia coli BL21(DE3) transduced with plasmid pRSET-B tdTomato (Tsien Laboratory, University of California, San Diego), extracted by cell-lysis and isolated by centrifugation and immobilized metal affinity chromatography. Fluorescence self-quenching Solutions of eGFP and pyrromethene dye (PM556, Exciton, USA) with different concentrations were filled into a 10-μm thick glass cell. The solid-state samples were 2.5 μm thick. Samples were excited in front-face configuration with a 473-nm laser. The fluorescence intensity was also recorded front-face using a 14-bit CCD detector (Andor), adjusting exposure time to maintain linear response. Depletion of the excitation light in highly concentrated samples is accounted for by quoting the effective fluorescence intensity ( I c ) instead of quoting the directly measured intensity ( I ). where c is the concentration of the sample, ε is the absorption coefficient at 473 nm and L =10 μm is the thickness of the glass cell. Due to the thin sample cell, depletion can be neglected for c <1 mmol l −1 . ASE measurements A thin film of eGFP was fabricated by spin-coating 200 μl of a 1 mmol l −1 solution onto a 1′ × 1′ glass substrate at 1,000 r.p.m. The film was excited by focusing the expanded output of an OPO (Quanta Ray MOPO-700, Spectra Physics; pulse duration, ~5 ns; tuned to 485 nm) to a stripe using a cylindrical lens. The stripe length was adjusted (to 3 mm unless stated otherwise) using a linear aperture mounted on a micro-translation stage. The pulse energy was adjusted by calibrated optical density filters. The emission was analysed by a spectrometer with a cooled CCD detector (Andor). Protein VCSELs Optical pumping was provided by focusing the output of a 473-nm microchip laser (RPMC Lasers) into the cavity with a × 4 objective. The output was again collected with a spectrometer. Each data point in the input–output characteristics represents the average over 500 excitation pulses. Protein ring lasers Protein rings were fabricated by pipetting 0.5-μl droplets of eGFP solution (100 μmol l −1 ) onto a silicon wafer coated with a 4-μm-thick spacer layer of Cytop (Asahi Glass Co., n =1.34). The droplets were left to dry at room temperature under ambient conditions. All-optical protein ring sensors Substrates were fabricated by melt-pressing poly(lactic acid) at 180 °C into 200-μm thick films. Films were cut into 5 × 10 mm 2 pieces, protein rings were deposited by pipetting and a multimode optical fibre was glued to the edge of the film. The opposite end of the fibre was coupled to a blue LED ( λ max =455 nm, FWHM=15 nm) and a spectrometer using a free space dichroic beam splitter. FRET lasers Solutions of eGFP and tdTomato were mixed at different ratios and vortexed to ensure complete mixing. Solid-state samples were obtained by pipetting onto Cytop-coated Si-wafers or onto DBR mirrors with a maximum reflectivity at 630 nm. Solution-based lasers comprised two concave DBR mirrors (peak reflectivity, 630 nm) separated by ~7 mm. Förster radii were calculated from measured emission and absorption spectra of donor and acceptor using the method described in ref. 44 . How to cite this article: Gather, M. C. and Yun, S. H. Bio-optimized energy transfer in densely packed fluorescent protein enables near-maximal luminescence and solid-state lasers. Nat. Commun. 5:5722 doi: 10.1038/ncomms6722 (2014).